Structural phase transitions in two-dimensional Mo- and W-dichalcogenide monolayers Mo- and W-dichalcogenide compounds have a two-dimensional monolayer form that differs from graphene in an important respect: it can potentially have more than one crystal structure. Some of these monolayers exhibit tantalizing hints of a poorly understood structural metal-to-insulator transition with the possibility of long metastable lifetimes. If controllable, such a transition could bring an exciting new application space to monolayer materials beyond graphene. Here we discover that mechanical deformations provide a route to switching thermodynamic stability between a semiconducting and a metallic crystal structure in these monolayer materials. Based on state-of-the-art density functional and hybrid Hartree–Fock/density functional calculations including vibrational energy corrections, we discover that MoTe 2 is an excellent candidate phase change material. We identify a range from 0.3 to 3% for the tensile strains required to transform MoTe 2 under uniaxial conditions at room temperature. The potential for mechanical phase transitions is predicted for all six studied compounds. The discovery of a mechanical exfoliation method [1] for two-dimensional (2D) crystals has led to the discovery of fundamentally new physics, and it was a watershed in the search for the materials that will take the centre stage in tomorrow’s technology. Among the layered crystals amenable to isolation of atomically thin monolayers is a large family of transition metal dichalcogenides (TMDs) having the chemical formula MX 2 , where M is some transition metal and X stands for S, Se or Te. The mostly semiconducting [2] subset of TMDs where the transition metal M is Mo or W (both in group VI) has received the greatest amount of attention in the pursuit of applications, including ultrathin flexible electronics [2] , [3] , [4] , [5] , [6] , [7] , [8] and valleytronics [9] , [10] . In an energy context, these materials hold promise as hydrogen evolution catalysts when certain features are exposed to the reacting environment [11] , [12] , [13] , [14] , [15] , [16] . A special but often overlooked feature of group VI TMD monolayers is that they have more than one possible 2D crystal structure. This polymorphism sets group VI TMD monolayers apart from other 2D materials such as graphene and hexagonal BN [17] , [18] , [19] . Intriguingly, one of these structural phases is semiconducting, whereas the others are metallic, unlike in the case of group V TMDs, where electrically activated metal-to-metal structural phase transitions have been demonstrated in multilayer TaS 2 (ref. 20 ) and TaSe 2 (ref. 21 ). It has been suggested that coexistence of metallic and semiconducting regions on a monolithic MX 2 nanosheet can be used to make electronic devices [18] , and metallic regions have been associated with catalytic activity leading to hydrogen evolution [12] , [16] , [22] . Moreover, materials with dynamic metal-to-insulator transitions close to ambient conditions are exceedingly rare and worth pursuing because of their nonvolatile information storage potential. Because the TMD metal-to-insulator transition is structural in nature, considerable metastability and hysteresis are expected to occur. This useful feature is absent in approaches where band gap closure is achieved by (and conditional on) large macroscopic strains to a fixed and normally semiconducting TMD structural phase [23] . Phase transitions are even more exciting in monolayers, which also provide opportunities for flexible, low-power and transparent electronic devices. Despite the clear motivation for doing so, it has thus far proven to be challenging to transform semiconducting MX 2 compounds to a stable metallic phase. A process of lithium-based chemical exfoliation of bulk crystals has been shown to be a successful route to obtain a metastable metallic phase of the group VI TMDs [18] , [24] , [25] , [26] . It is, however, uncertain that this phase would persist under all realistic operating conditions, and reversible switching is not demonstrated in this case. One would like to know under what thermodynamic conditions (if any) metallic phases of TMDs are expected to be stable rather than just metastable. This insight would point in a direction of dynamic phase switching and large-area synthesis of the elusive metallic phase using standard chemical growth techniques, such as chemical vapour deposition. Chemical growth techniques are an area of rapid progress in recent years [27] , [28] , [29] , [30] , [31] , [32] . One would furthermore like to know what TMD compounds are nearest to the phase boundaries at ambient conditions, and therefore most amenable to applications involving transformations between phases or mixed-phase regimes. Here we use density functional theory (DFT) and DFT-based methods to determine the phase diagrams of TMD monolayers as a function of strain. We find that equibiaxial tensile strains of 10–15% are required to observe the metallic phase for most TMDs, but MoTe 2 may transform under considerably less tensile strain, <1.5% under appropriate constraints. We further discover that mixed-phase regimes can be thermodynamically stable under certain thermodynamic constraints that are readily achievable in the laboratory. Monolayer crystal structures Under ambient conditions, all group VI TMDs (except WTe 2 ) are reported to exist in a layered bulk crystal structure composed of monolayers wherein the X atoms are in trigonal prismatic coordination around the M atoms [17] . The atomic stacking sequence within a single XMX monolayer is βAβ. In keeping with prior literature, we will refer to this as the 2H phase, even though the prefix ‘2’ is irrelevant in monolayers because it refers to a bulk stacking mode. Group VI MX 2 monolayers in the 2H structure are semiconducting with band gaps between 1 and 2 eV (refs 2 , 33 , 34 ). 2H TMDs are promising semiconductors for flexible electronics applications [2] , [3] , [4] , [5] , [6] , [7] , [8] . The 2H structure gives rise to metallic edge states that are associated with electrocatalytic activity [11] . The primitive unit cell of the 2H phase is hexagonal. For reasons of consistency between different phases, our calculations on 2H use a non-primitive rectangular unit cell whose axes align with zigzag and armchair directions of the structure. These special axes can be experimentally identified using second harmonic generation [35] , [36] , and possibly also using the intrinsic piezoelectricity predicted to exist in these materials [37] . 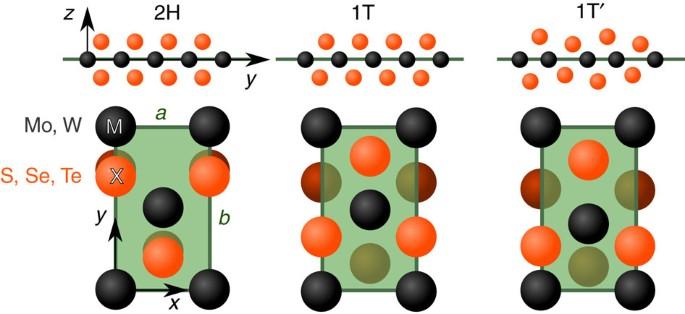Figure 1: The three crystalline phases of 2D group VI TMDs. Each can be represented in a rectangular unit cell with dimensionsa×b. All three phases consist of a metal (Mo/W) atom layer sandwiched between two chalcogenide (S/Se/Te) layers. The semiconducting 2H phase is often referred to as the trigonal prismatic structure, and the metallic 1T and 1T′ are called octahedral and distorted octahedral, respectively. The 1T′ phase can be thought of as 1T after a symmetry-reducing distortion. Figure 1 shows the 2H structure within a rectangular unit cell having lattice constants a and b . Figure 1: The three crystalline phases of 2D group VI TMDs. Each can be represented in a rectangular unit cell with dimensions a × b . All three phases consist of a metal (Mo/W) atom layer sandwiched between two chalcogenide (S/Se/Te) layers. The semiconducting 2H phase is often referred to as the trigonal prismatic structure, and the metallic 1T and 1T′ are called octahedral and distorted octahedral, respectively. The 1T′ phase can be thought of as 1T after a symmetry-reducing distortion. Full size image When one of the 2H structure’s X layers is shifted (for instance, βAβ→βAγ), the X atoms are in octahedral coordination around the M atoms, and the crystal becomes metallic. This phase is referred to as 1T and is observed in group IV and group V TMD compounds (for example, TiS 2 and TaSe 2 (ref. 17 )). Its atomic structure is also shown in Fig. 1 . We have calculated the atomic vibrational normal modes (Г-phonons) within the relaxed rectangular 1T unit cell of all six group VI TMDs. In all cases, one of the optical phonon modes has an imaginary vibrational frequency. This result asserts that the high-symmetry 1T structure is unstable (saddle point in 18D atomic potential energy surface), at least in the absence of external stabilizing influences. The group VI TMDs do have a stable metallic structure with octahedral-like M–X coordination. This lower-symmetry phase, which we will refer to as 1T′, is a distorted version of the 1T structure [12] , [17] , [38] . This phase has recently been shown to enhance electrocatalytic activity in WS 2 (ref. 12 ). A rectangular (as well as primitive) 1T′ unit cell is displayed in Fig. 1 . The 1T′ phase is observed in WTe 2 under ambient conditions [17] , MoTe 2 at high temperature [39] and as a metastable phase in instances of chemically exfoliated [18] and restacked [38] MX 2 monolayers. 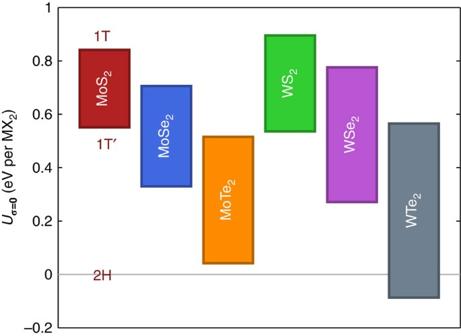Figure 2: Ground-state energy differences between monolayer phases of the six studied materials. The energyUis given per formula unit MX2for the 2H, 1T′ and 1T phases. Its value is computed at the equilibrium (zero stress,σ) lattice parameters for each phase. Becauseσ=0, these values forUare equivalent to the enthalphyH. Vibrational energy is not included in these values. Phase energetics in the absence of mechanical stress Figure 2 shows the calculated equilibrium (that is, stress-free) relative energies of the phases (2H, 1T and 1T′) of the group VI MX 2 monolayer materials. These values are calculated using DFT under the generalized gradient approximation (GGA) for electronic exchange and correlation effects, using the Perdew–Burke–Ernzerhof [40] (PBE) functional. The results are consistent with the experimental observation for bulk crystals that only WTe 2 is 1T′ under ambient conditions [17] . It is also evident from these data that the energy associated with the 1T to 1T′ relaxation is considerable: several tenths of an eV per MX 2 formula unit. The three phases’ equilibrium lattice constants and energies are tabulated in Supplementary Table 1 . Figure 2: Ground-state energy differences between monolayer phases of the six studied materials. The energy U is given per formula unit MX 2 for the 2H, 1T′ and 1T phases. Its value is computed at the equilibrium (zero stress, σ ) lattice parameters for each phase. Because σ = 0 , these values for U are equivalent to the enthalphy H . Vibrational energy is not included in these values. Full size image Phase energetics under biaxial strain Thermodynamics asserts that a system will seek to minimize whichever thermodynamic potential is appropriate for the prevailing mechanical and thermal boundary conditions [41] . The simplest example of such a thermodynamic potential is the internal energy U . In the low-temperature limit, any system will seek to minimize U when it is constrained to a given shape. Under these conditions, an MX 2 monolayer constrained to be described by a rectangular unit cell with dimensions a × b is expected to be in the lower- U phase for those values of a and b . Experimentally, relevant phase diagrams of monolayers differ from those of bulk materials at high pressure in at least one important respect: the monolayer can be mechanically coupled to a substrate with friction, enabling the independent control of a and b lattice parameters ( Fig. 3 ). Another key distinction is that large elastic deformations in monolayers can be reached through tensile strain [42] , [43] , whereas large elastic deformations in most bulk materials are accessible only under compression. Large compressive stresses are problematic in TMD monolayer materials due to the spontaneous ripple formation that has been studied in MoS 2 (refs 44 , 45 ). 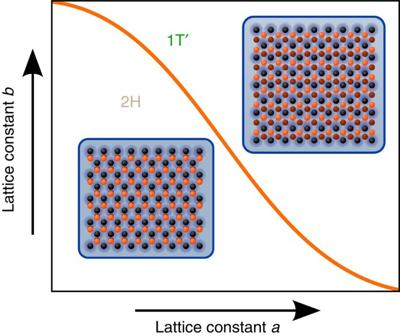Figure 3: Substrate-based application of strain to a TMD monolayer. One way in which the lattice parametersaandbof an MX2monolayer may be tuned is by virtue of an underlying substrate (shown in blue). Because the substrate and the monolayer have a preferred crystallographic alignment, the deformation of the substrate can be transferred to the TMD monolayer. If the values of the lattice constantsaandbaffect which of the phases is thermodynamically stable, the application of strain (or chemical growth of the monolayer on a strained substrate) can be used to select a particular phase. Figure 3: Substrate-based application of strain to a TMD monolayer. One way in which the lattice parameters a and b of an MX 2 monolayer may be tuned is by virtue of an underlying substrate (shown in blue). Because the substrate and the monolayer have a preferred crystallographic alignment, the deformation of the substrate can be transferred to the TMD monolayer. If the values of the lattice constants a and b affect which of the phases is thermodynamically stable, the application of strain (or chemical growth of the monolayer on a strained substrate) can be used to select a particular phase. Full size image For the six group VI MX 2 monolayers, we use GGA–DFT to calculate the energies U ( a , b ) of the three monolayer crystal structures on a 7 × 7 grid in ( a , b ) space, giving a total of 49 points of ( a , b )-values around the minimum-energy equilibrium lattice constants a 0 and b 0 (listed in Supplementary Table 1 ). U is obtained after allowing the ions to relax their positions within each unit cell. Intermediate values for each phases’ U ( a , b ) are subsequently approximated using the Lagrange [46] interpolation method: Lagrange interpolation is chosen because it contains no physical assumptions about the shape of the U ( a , b ) energy surface over a large range of tensile and compressive strains. It also greatly facilitates the approximation of local derivatives (which we need later) without suffering from conditioning problems found in other high-order polynomial methods. Using this approach, we discover that the 2H and 1T′ U ( a , b ) energy surfaces intersect for sufficiently large strains. 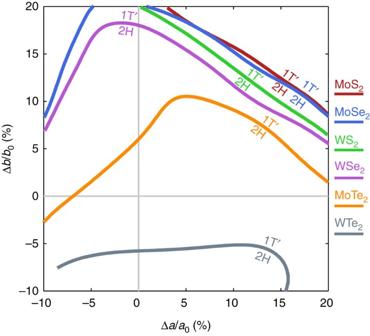Figure 4: Intersection contours of the 2H and 1T′ energy surfaces when varying the rectangular lattice constantsaandb. The lattice constantsaandbare represented as percent engineering strains, normalized over the equilibrium lattice constantsa0andb0of the lowest energy structure (2H in all cases except WTe2). The lower-energy (that is, lower-U) phase is labelled on each side of the contours. Figure 4 shows the contours that follow the intersection of the 2H and 1T′ energy in ( a , b ) space. The changes in a and b required to change the relative energies U of the 2H and 1T′ phase range from 13% (MoS 2 ) to 3% (MoTe 2 ). Because many bulk materials begin to dissipate strain energy through fracture or dislocations at strains on the order of 0.1% (roughly 10 −5 eV per atom), these threshold strains may at first appear to be prohibitively large. However, it has been experimentally demonstrated that monolayer TMDs are exceedingly strong: Bertolazzi et al. [42] have performed atomic force microscopy (AFM) experiments where 2H-MoS 2 monolayers are shown to reversibly withstand in-plane tensile stresses up to 15 Nm −1 , corresponding to ~10% of the material’s in-plane Young’s modulus. Such deformations correspond to an elastic energy of order 0.1 eV per atom. From the local derivatives of the 2H phase’s U ( a , b ) at the equibiaxial transition strain, we find that the 2H stresses (in Nm −1 ) at this point are 12.8 (MoS 2 ), 10.8 (MoSe 2 ), 6.9 (MoTe 2 ), 13.6 (WS 2 ) and 10.5 (WSe 2 ). This suggests the possibility that a transition between 2H and 1T′ might be observable below but near the breaking threshold. Figure 4: Intersection contours of the 2H and 1T′ energy surfaces when varying the rectangular lattice constants a and b . The lattice constants a and b are represented as percent engineering strains, normalized over the equilibrium lattice constants a 0 and b 0 of the lowest energy structure (2H in all cases except WTe 2 ). The lower-energy (that is, lower- U ) phase is labelled on each side of the contours. Full size image From Fig. 4 , we can also see that WTe 2 , which is usually in the 1T′ phase, can be pushed into a 2H regime under compression, which is complementary to all the other cases where one would go from 2H to 1T′ through tension. While this is interesting, we will not focus on it since in-plane compression in monolayer WTe 2 may be experimentally challenging to achieve without incurring any buckling response. From the contours in Fig. 4 , it is also apparent that a 2H-1T′ transition might be most easily accessible in MoTe 2 under tension along the b axis. The remainder of the Results section will find that the predicted phase boundary for MoTe 2 moves even closer to ambient conditions when including thermal effects, more advanced treatments of electronic exchange and correlation, and by generalizing the governing thermodynamic constraints beyond the case of fixed lattice constants. Thermal corrections in MoTe 2 The data shown in Figs 2 and 4 derive from the DFT-calculated potential energy U = U crystal , and therefore omit the vibrational component of free energy. This vibrational component can be important when the energy difference between phases is <0.1 eV, on the order of k B T . Figure 2 shows that the 1T′-2H energy offset thus calculated for MoTe 2 is sufficiently small (43 meV) such that vibrational effects could have a role in the energetic ordering of phases. For a temperature-controlled experiment, the Helmholtz free energy A ( a , b , T ) replaces U ( a , b ) as the relevant thermodynamic potential. We perform this calculation for MoTe 2 by treating the DFT-calculated vibrational normal modes as quantum mechanical harmonic oscillators [47] . We shall see that these effects in MoTe 2 have a considerable impact, even in the idealized T →0 K case because of contributions from the vibrational zero-point energy, which can be regarded as a manifestation of the partially wavelike nature of the atomic nuclei. In the case of 2H- and 1T′-MoTe 2 , we calculate a temperature-dependent vibrational free-energy correction based on the frequency spectrum of the 15 nonzero Г-point phonons belonging to the rectangular cell of each phase. These phonon frequencies are obtained by applying linear-response theory to the forces in perturbed unit cell configurations for all 7 × 7 ( a , b ) grid points. We then add the quasi-harmonic vibrational free-energy correction A vib = U vib – TS vib to the potential energy U crystal : Since this approach samples 15 discrete values of ω i at Г, it does not take into account the full dispersion of phonon frequencies for arbitrary wave vectors in the Brillouin zone. Large supercell calculations that sample the vibrational spectrum more finely (up to 159 values of ω i in a 3 × 3 supercell) reveal that the use of 15 phonons in equation (2) leads to errors under 3 meV per MoTe 2 formula unit when comparing 2H and 1T′ free energies ( Supplementary Fig. 1 ). This error is significantly smaller than the 1T′-2H’ U crystal energy difference of 43 meV. Proceeding with the results of equation (2), the Lagrange interpolation procedure is carried out again at intermediate values of a and b . The top three curves in Fig. 5 show that the vibrational correction A vib moves the PBE-calculated ( a , b )-space free-energy crossing in MoTe 2 to smaller strains. Indeed, a 0-K zero-point free-energy correction lowers the threshold strain by up to 0.01 in some regions, and increasing the temperature from 0 to 300 K produces another shift of up to 0.02 in the same regions. 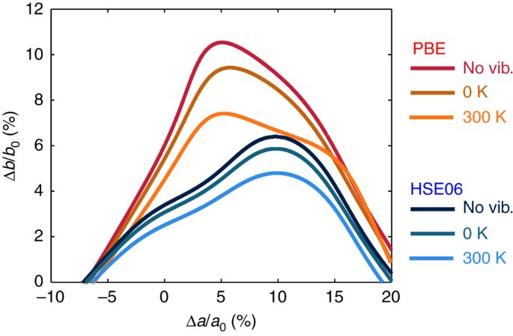Figure 5: Vibrational effects and hybrid functionals in MoTe2. This figure shows the intersections of the MoTe22H and 1T′ free energiesA(a,b,T) using different treatments of vibrational (vib.) effects and two exchange–correlation functionals. The top curve (GGA–DFT, no vibrational effects) corresponds to the MoTe2countour inFig. 4. Inclusion of vibrational free energy at 0 K (that is, only the vibrational zero-point energy) and at 300 K shifts the onset of the 1T′ regime closer to the origin. It can also be seen from this figure that the use of the HSE06 DFT/Hartree–Fock functional in lieu of PBE has a similar effect. Figure 5: Vibrational effects and hybrid functionals in MoTe 2 . This figure shows the intersections of the MoTe 2 2H and 1T′ free energies A ( a , b , T ) using different treatments of vibrational (vib.) effects and two exchange–correlation functionals. The top curve (GGA–DFT, no vibrational effects) corresponds to the MoTe 2 countour in Fig. 4 . Inclusion of vibrational free energy at 0 K (that is, only the vibrational zero-point energy) and at 300 K shifts the onset of the 1T′ regime closer to the origin. It can also be seen from this figure that the use of the HSE06 DFT/Hartree–Fock functional in lieu of PBE has a similar effect. Full size image Kinetic aspects of the MoTe 2 phase transition Thus far, our purely thermodynamic analysis does not provide information regarding the timescales required to observe a transition between the 2H and the 1T′ phase. Experimental observation of a thermodynamically allowed transformation might not be feasible if a large kinetic barrier renders it inaccessible. A Climbing-Image Nudged Elastic Band [48] calculation within GGA–DFT reveals a 2H-1T′ energy barrier of 0.88 eV per formula unit in MoTe 2 at the equilibrium lattice constants of the 2H phase. In the Arrhenius kinetics picture with a characteristic frequency of 10 THz, the timescale associated with this barrier is 50 s at room temperature. Although other factors such as interfaces, substrate, temperature, strain and impurities are likely to alter the transformation kinetics, this timescale suggests that this transformation is likely to be observable in the room temperature laboratory. Hybrid functional applied to MoTe 2 Like many contemporary computational materials studies, our results presented thus far rely heavily on the generalized gradient PBE [40] functional for electronic exchange and correlation effects. The development of new exchange–correlation functionals is a highly active field, and a Hybrid PBE/Hartree–Fock approach known as the Heyd–Scuseria–Ernzerhof HSE06 (ref. 49 ) functional has recently shown superior agreement with experimental results in structural metal–insulator transition phase boundaries in Si [50] . To explore how HSE06- and PBE-based predictions differ in a MoTe 2 context, we recalculate the U crystal component of equation (2) using the HSE06 functional on the 7 × 7 grid of PBE-relaxed geometries. The HSE06-based phonon spectrum is not recalculated for this work because of the formidable computational demands presently posed by high-quality HSE06 calculations. Instead, the PBE-calculated frequencies are reintroduced on top of the HSE06-calculated U crystal . The bottom three curves in Fig. 5 show that use of the HSE06-calculated U crystal brings the 2H-1T′ threshold strains even closer to the origin. At 300 K, the transition is predicted to be within 2% strain of the equilibrium 2H lattice constants. Alternative thermodynamic constraints Some careful consideration of the relevant thermodynamic constraints is warranted here for the case of monolayers. The thermodynamic constraint of fixed lattice constants used in Figs 4 and 5 is an unusual one (different from constant volume or area) that is perhaps most applicable when crystallographic coherence is maintained with a strongly binding substrate. At some fixed temperature T , the Helmholtz free energy A ( a , b , T ) is the thermodynamic potential whose minimization determines which crystal phase (or coexistence of phases) will exist in a crystal possessing a rectangular unit cell with dimensions a × b . However, this fixed-cell constraint certainly need not apply when friction with the substrate is weak, or when the monolayer is freely suspended. In analogy with the important distinction between constant-pressure and constant volume experiments in bulk materials, we now show how to generalize our MoTe 2 results to other thermodynamic constraints with stable two-phase coexistence regions. Perhaps the simplest thermodynamic constraint occurs when both in-plane principal tensions are equal, such that σ xx = σ yy . This isotropic-tension condition is analogous to the isotropic constant-pressure case in three dimensions. The natural thermodynamic potential governing this isotropic-load system (that is, the potential that is minimized) is a ‘hydrostatic’ Gibbs free energy G hydro , where the surface tensions σ xx = σ yy ≡ σ and σ xy =0: The previously independent variables ( a , b , T ) used in A = A ( a , b , T ) are now a function of (σ, T ) through the definition of a 2D hydrostatic contour { a , b }={ a (σ, T ),b(σ, T )}. This contour is determined directly from the interpolated A ( a , b , T ) surface and its local derivatives (for example, using σ xx =(1/ b )∂ A /∂ a ). Another physically relevant constraint is that of constant area. This is closely related to a constant volume constraint for bulk materials. Such a constraint can lead to mixed-phase regimes. Constant area is a macroscopic constraint that might be applicable when the edges of a freely suspended monolayer are clamped in place to fix the area, independent of stress. A very useful constraint applies when one of the principal tensions is zero, for example, when σ xx = σ xy =0 and σ yy is nonzero. This condition might hold for a ribbon suspended over a trench. Considering the 2H-1T′ energy landscape in Fig. 4 , it would appear promising to apply a uniaxial stress along the b axis of MoTe 2 in order to observe a phase transition. We therefore study a system that is subjected to a specified uniaxial-load F y =∂ A /∂ b along the crystal’s special y axis, whereas the x -face is treated as a free surface (that is, ∂ A /∂ a =0). Applying the appropriate Legendre transform to A for this case yields another Gibbs-like free energy G y that acts as the governing thermodynamic potential. In our data, the independent variables ( F y , T ) can be mapped to a uniaxial-load contour { a , b }={ a ( F y , T ), b ( F y , T )}, derived from the interpolated A ( a , b , T ) surface and its local derivatives. This approach carries the microscopic assumption that both the 2H and the 1T′ phases’ b axes point in the y direction. A closely related case is that of fixed macroscopic uniaxial strain. In the macroscopic uniaxial-strain case, one assumes that the lattice constant a remains fixed at the same value for both phases, such that strain occurs along both phases’ b axis. Macroscopic uniaxial strain allows for two-phase coexistence regimes with crystallographic coherence between the 2H and 1T′ phase. Macroscopic uniaxial strain is also relevant if the substrate–TMD interaction is strongly anisotropic. The strain ε yy =‹ b ›/ b 0 −1 is termed macroscopic because b is the weighted average over two different lattice constants ‹ b › when strained 2H and 1T′ phases coexist. In an experiment, changes in b are proportional to the macroscopic extension of the sample. Additional thermodynamic ensembles may be applicable for monolayers. For example, when a monolayer is weakly bound to a substrate with friction, the atoms are allowed to move to some limited extent and restricted by contact with the surface. The thermodynamic potential of the TMD monolayer will be some intermediate case between the constant-force case (applicable to a frictionless substrate) and the fixed-( a , b ) case where friction is large enough to inhibit significant movement of the metal atoms. Alternative thermodynamic constraints applied to MoTe 2 Both the hydrostatic and uniaxial-load contours are displayed in Fig. 6a (PBE-calculated U crystal ) and Fig. 6b (HSE06-calculated U crystal ). When increasing F y or σ , at some point the Gibbs free energies of the 2H and 1T′ phases cross. When that happens, the resulting phase transition can be seen as a discontinuous jump in ( a,b )-space from the 2H to the 1T′ contour. It is interesting to note that at precisely this transition load, any mixed-phase coexistence of both phases ranging from 100% 2H to 100% 1T′ is thermodynamically stable. Figure 7 illustrates the general concept of mixed-phase regimes when a monolayer is progressively tensioned, for example, by increasing F y or ‹ b › (for the uniaxial stress/strain case), or by increasing hydrostatic stress σ or the unit cell area ab . 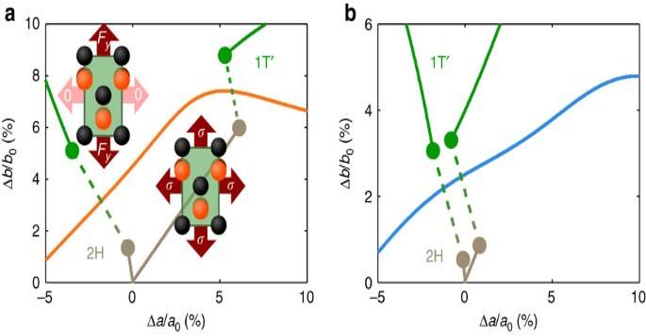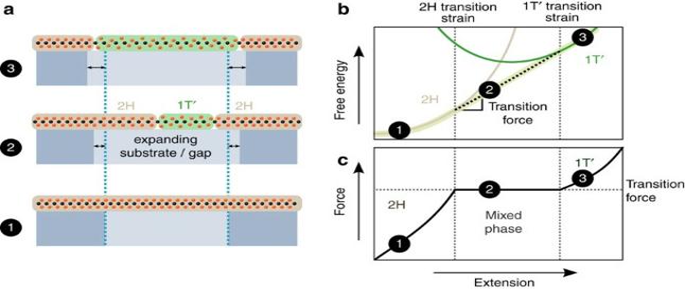Figure 7: Phase coexistence under an applied force or extension. A tensile mechanical deformation (for example, hydrostatic, uniaxial load or uniaxial strain) expands a region of the TMD monolayer. This strained region can be freely suspended or locally sliding over a low-friction substrate, as shown ina. The 2H/1T′ Helmholtz free energy landscapebis traversed in this process. In step 1, the 2H phase deforms elastically and no phase transition is observed. Beyond some critical strain in step 2, the lowest free-energy path is a common tangent between the 2H and 1T′ energy surfaces, manifesting a coexistence regime where both phases are coexisting in mechanical equilibrium. If the experimental setup is such that the extension is controlled (for example, using a stiff AFM probe), this region is observed as a plateau in the applied forcec. At the strain level of step 3, the lowest energy phase is composed of 100% 1T′, completing the mechanically induced phase transition. Figure 6: Load-specific trajectories and transitions of MoTe2at 300 K. Panelauses the PBE functional to calculate the crystal energy, whereas the HSE06 functional is used inb. Starting at their stress-free 2H equilibrium valuesa0andb0, the lattice constantsaandbevolve in response to progressive application of a uniaxial-load (Fy) or a ‘hydrostatic’ isotropic tension (σ). At a certain load, the 2H and 1T′ thermodynamic potentials cross. When this transition occurs, the lattice constants jump from their 2H to their 1T′ values. A coexistence regime is expected to exist in the dashed regions, where increasing theblattice constant while keepingFx=0 (uniaxial load) or increasing the areaabunder hydrostatic conditions can yield regions of 2H and 1T′ in the monolayer. Although the solid trajectories appear to be mostly rectilinear, they represent an aggregate of finely sampled data points travelling along the Lagrange interpolation surface. Figure 6: Load-specific trajectories and transitions of MoTe 2 at 300 K. Panel a uses the PBE functional to calculate the crystal energy, whereas the HSE06 functional is used in b . Starting at their stress-free 2H equilibrium values a 0 and b 0 , the lattice constants a and b evolve in response to progressive application of a uniaxial-load ( F y ) or a ‘hydrostatic’ isotropic tension ( σ ). At a certain load, the 2H and 1T′ thermodynamic potentials cross. When this transition occurs, the lattice constants jump from their 2H to their 1T′ values. A coexistence regime is expected to exist in the dashed regions, where increasing the b lattice constant while keeping F x =0 (uniaxial load) or increasing the area ab under hydrostatic conditions can yield regions of 2H and 1T′ in the monolayer. Although the solid trajectories appear to be mostly rectilinear, they represent an aggregate of finely sampled data points travelling along the Lagrange interpolation surface. Full size image Figure 7: Phase coexistence under an applied force or extension. A tensile mechanical deformation (for example, hydrostatic, uniaxial load or uniaxial strain) expands a region of the TMD monolayer. This strained region can be freely suspended or locally sliding over a low-friction substrate, as shown in a . The 2H/1T′ Helmholtz free energy landscape b is traversed in this process. In step 1, the 2H phase deforms elastically and no phase transition is observed. Beyond some critical strain in step 2, the lowest free-energy path is a common tangent between the 2H and 1T′ energy surfaces, manifesting a coexistence regime where both phases are coexisting in mechanical equilibrium. If the experimental setup is such that the extension is controlled (for example, using a stiff AFM probe), this region is observed as a plateau in the applied force c . At the strain level of step 3, the lowest energy phase is composed of 100% 1T′, completing the mechanically induced phase transition. Full size image In the uniaxial-load case for MoTe 2 , the calculated strains ε yy = b / b 0 –1 required to enter the 2H end of this transition regime are shown in Fig. 8a . It is striking that the choice of exchange–correlation functional and the treatment of atomic vibrations have a large impact on this number: ε yy ranging from 0.5% (HSE06, 300 K) to 2.4% (PBE, no vibrational free energy). 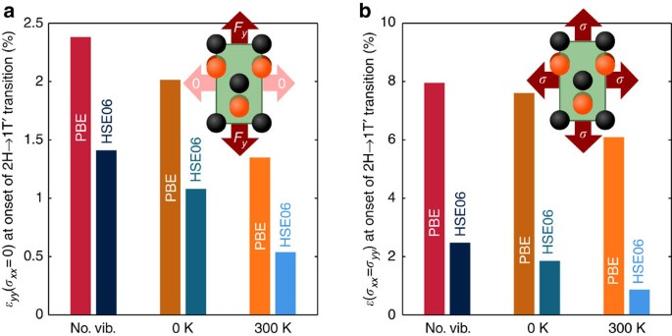Figure 8: Strain at onset of load-specific 2H to 1T′ transitions in MoTe2. This figure is closely related toFig. 6. The application of a uniaxial load or isotropic tension affects the relative thermodynamic potential of the 2H and 1T′ phases. The strains plotted here are the predicted maximum strains in 2H before transformation to 1T′ is thermodynamically possible. The chart inashows the threshold strainsεyy=Δb/b0under uniaxial load. The equibiaxial threshold strainsε=Δa/a0=Δb/b0under isotropic tension are shown inb. It can be seen that the choice of exchange–correlation functional as well as the treatment of vibrational (vib.) free energy have a marked effect on these strain values. Figure 8b shows that the strain on the 2H end of the hydrostatic transition is similarly sensitive to temperature and electronic exchange–correlation functional. The discrepancy between PBE and HSE06 shows a clear path towards experimentally addressing the question of which functional is better suited for 2D materials studies. Figure 8: Strain at onset of load-specific 2H to 1T′ transitions in MoTe 2 . This figure is closely related to Fig. 6 . The application of a uniaxial load or isotropic tension affects the relative thermodynamic potential of the 2H and 1T′ phases. The strains plotted here are the predicted maximum strains in 2H before transformation to 1T′ is thermodynamically possible. The chart in a shows the threshold strains ε yy = Δb / b 0 under uniaxial load. The equibiaxial threshold strains ε = Δa / a 0 = Δb / b 0 under isotropic tension are shown in b . It can be seen that the choice of exchange–correlation functional as well as the treatment of vibrational (vib.) free energy have a marked effect on these strain values. Full size image The accuracy of these predictions of small transition strains based on 2D interpolation is validated using additional calculations in the case of MoTe 2 . We run a 10 × 10 grid of PBE, phonon and HSE06 calculations in a region in ( a , b )-space with axial strains ranging from −5 to 10%. This new data set is three times as fine as the 7 × 7 grid and also includes PBE-calculated phonons. Coexistence regimes are extracted from a series of 1D fits on this refined grid, as illustrated in Supplementary Fig. 2 . The typical difference between uniaxial-load transition strains from this approach and the equivalent strains from the 2D Lagrange-interpolating method used throughout the main text is 0.002 for HSE06 and 0.005 for PBE ( Supplementary Fig. 3 ). In the case of macroscopic uniaxial strain at 300 K (not shown in Fig. 8 ), the HSE06 functional predicts an onset of the coexistence regime at 1.6% strain, whereas PBE predicts 3.0%. These strains are obtained from 1D cubic fits (illustrated in Supplementary Fig. 4 ) on the refined 10 × 10 grid of DFT-calculated energies, at fixed lattice constant a =3.550 Å and varying b . Supplementary Figure 5 summarizes all uniaxial-load and uniaxial-strain results based on this 10 × 10 grid. Recent calculations and AFM experiments [43] have demonstrated that a MoS 2 monolayer can be subjected to 20% equibiaxial strain. In these experiments, a pre-tensioned MoS 2 sheet is pushed into a circular cavity by means of an AFM probe. These experiments report no evidence of a phase transition, but do report the presence of sufficiently large equibiaxial deformations ( Fig. 4 ) in the small region under the AFM tip. The indentation timescale (~1 s) may be too short to observe a transition, perhaps even more so because the AFM tip may increase the 2H-1T′ transition energy barrier. On the other hand, this reference [43] does note that the majority of samples show a significant force–displacement hysteresis that is attributed to slipping, but which might indicate a phase transition in light of the present study. Although widely studied today, MoS 2 monolayers are not ideally suited for phase transitions because MoS 2 has the greatest 1T′-2H energy difference of all group VI TMDs. 2H-1T′ structural phase transitions are closest to ambient conditions in the case of MoTe 2 . This property makes MoTe 2 more suitable for technological applications and is hoped to motivate further advances in telluride TMD growth techniques. In the case of MoTe 2 , certain classes of strain states are more likely to yield a phase transition than others. Based on the local characteristics of the MoTe 2 phases’ energy landscape, our research identifies the application of tension along the 2H phase b axis (armchair) as a fertile route to observing a phase transition. As a general trend, the deformations associated with this transition appear to be brought closer to zero with increasing temperature. At room temperature, we predict that the lowest strain ε yy needed to render the 1T′ phase stable lies between 0.3% (HSE06, uniaxial load) and 3% (PBE, uniaxial strain). The values quoted above are computed from the refined 10 × 10 grid of DFT calculations. We note that the calculated insulator-to-metal strains in monolayer MoTe 2 compare favourably with insulator-to-insulator transition strains reported for bulk VO 2 (ref. 51 ), which has no known 2D form. Stress and strain could be applied to a TMD monolayer via deformation of a flexible substrate. Another approach, which might yield more quantitative evidence of the transition process, is to perform an experiment where an AFM probe pushes down a freely suspended MoTe 2 monolayer with its armchair axis pointing across a trench as shown in Fig. 7 . As with all DFT calculations, the equilibrium 2H and 1T′ lattice constants calculated in this work are expected to exhibit discrepancies with experimental lattice constants on the order of 1%. For example, our DFT-calculated 2H-MoS 2 monolayer lattice constant a of 3.18 Å is within 2% of measured values from 3.1 to 3.2 Å in chemically grown MoS 2 (ref. 27 ). A discrepancy in the actual location of energy minima in ( a , b )-space will offset the strains needed to achieve phase transitions by a similar amount in percentage points. The error in our calculated MoTe 2 lattice constants is unknown because no experimental lattice constants for 2H and 1T′ monolayers have been reported (to the best of our knowledge). Since our research compares crystal structures having the same chemical composition, we believe that the DFT error in lattice constants will be systematic across different phases, leading to a partial cancellation of errors in transition strains. Spontaneous ripple formation has been observed in MoS 2 (refs 44 , 45 ). These ripples (which are expected to exist in other TMDs as well) render the presence of significant compressive principal stresses in monolayers unlikely, reducing the possibility of observing a 1T′ to 2H transition in WTe 2 ( Fig. 4 ). Another technical consequence of pre-existing ripples is that some additional strain may be required before the mechanical stresses needed for a phase transition are present. The goal of this study is to investigate the possibility of a mechanical route to thermodynamically driven phase transformations between metal and semiconducting crystal structures in all group VI TMDs. Our results show that these mechanical transformations are in fact possible and most easily accessible in the case of MoTe 2 . With this information, we are optimistic that mechanically induced phase transitions can be achieved using flexible substrates, AFM techniques and other standard experimental approaches. This thorough understanding of phases and phase boundaries in TMD monolayers is a critical step towards building our understanding of the rich physics of 2D materials. Furthermore, the existence of multiple phases in monolayers is an exciting feature beyond graphene that undoubtedly has broad implications for electronic, Nanoelectromechanical systems (NEMS), thermal, energy and myriad other devices that can all benefit from the flexible, transparent nature of monolayers. Electronic structure calculations DFT and hybrid DFT calculations were performed using the Projector-Augmented Wave [52] , [53] pseudopotential implementation of the Vienna Ab Initio Simulation Package [54] , version 5.3.3. In the DFT calculations, electron exchange and correlation effects are described by the GGA functional of PBE [40] . Wave functions are expanded in a plane-wave basis set with a kinetic energy cutoff of 350 eV on an 18 × 18 × 1 Monkhorst-Pack [55] k-point grid using a Gaussian smearing of 50 meV. The convergence thresholds were 0.5 × 10 −6 eV per MX 2 and 0.5 × 10 −5 eV per MX 2 for electronic and ionic relaxations, respectively. The linear-response phonon calculations use an electronic threshold of 0.5 × 10 −8 eV per MX 2 . The Hybrid DFT calculations use the screened hybrid functional by Heyd, Scuseria and Ernzerhof [49] (HSE06). The electronic convergence threshold used for HSE06 calculations is 0.5 × 10 −5 eV/MX 2 . A total of 26 valence electrons per MX 2 are treated by HSE06, whereas the PBE calculations only treat 18 valence electrons. The computational cell height along the z-axis is 16 Å. Our computational unit cells of the 1T′ structure (shown in Fig. 1 ) belong to plane group pm . This plane group symmetry seems to be present or only very slightly broken in experimental data [17] , [38] . Our phonon analysis of this unit cell indicates that pm reflection symmetry is stable under ambient conditions. We recalculate 1T′ energies and intersection contours such as in Fig. 4 using the a × b cell but with broken symmetry ( p1 ). All except the highest-strain cases simply revert to the pm- symmetric case when the atoms are allowed to relax within the strained unit cell. We find that the 2H-1T′ intersection contours were virtually unaltered after allowing for broken pm -symmetry. Interpolation and fitting The Lagrange interpolation used to calculate forces and stresses for the hydrostatic and uniaxial-load trajectories was carried out on a 6 × 6 grid instead of the usual 7 × 7 grid, leaving out only the highest-strain points. In order to get uniaxial-load transition strains without Lagrange interpolation, we fit both 2H and 1T′ Helmholtz free energies along each ‘row’ i (having a fixed lattice constant b i ) in the 10 × 10 or 7 × 7 grid to a 1D cubic polynomial in the lattice constant a , A i ( b i , a ). The minima of A i ( b i , a ) are the points where ∂ A /∂ a = F x =0, satisfying the uniaxial-load constraint. For each phase, these minimum free energies are then re-fitted as a cubic function A ( b ). The resulting curves are used to compute the relevant Gibbs free energies, leading to new values for the uniaxial-load transition strains. The procedure is illustrated in Supplementary Fig. 2 . How to cite this article : Duerloo, K.-A.N. et al. Structural phase transitions in two-dimensional Mo- and W-dichalcogenide monolayers. Nat. Commun. 5:4214 doi: 10.1038/ncomms5214 (2014).